Subgenome-aware analyses suggest a reticulate allopolyploidization origin in threePapavergenomes 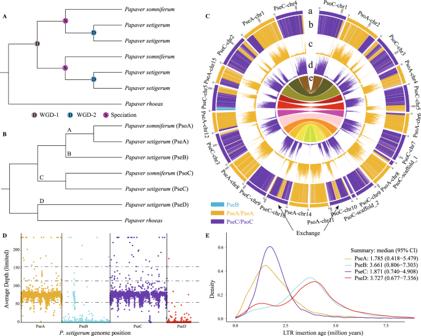Fig. 1: The origin and evolution of the subgenomes in the three studiedPapaverspecies. APhylogenomic relationships among the subgenomes assuming the whole-genome duplication (WGD) model of Yang et al.3.BTree topology recovered by gene trees, macro-synteny trees, and species/subgenome trees (see Supplementary Figs.4,5,8for details). The four subgenomes ofP. setigerumare designated PseA, PseB, PseC and PseD; the two subgenomes ofP. somniferumare designated PsoA and PsoC, and their ancestors are designatedA–D.CCircos plot of subgenome partitions ofP. somniferumandP. setigerumgenomes (more details in Supplementary Figs.6,7) indicates that PseA and PsoA, and PseC and PsoC share almost all subgenomic exchanges except a segment in PseC-chr5 that shows exchange with PseB. (a) Subgenome assignment of chromosomes based on thek-means algorithm. (b) Significant enrichment of subgenome-specifick-mers (subgenome partitions). Partitions with the same color as that of a subgenome indicates significant enrichment ofk-mers specific to that subgenome. The white areas are not significantly enriched. (c–d) Count (absolute) of each subgenome-specifick-mer set. (e) Homoeologous blocks between the two species. All statistics (b–d) were computed in sliding windows of 1 Mb. Exchanges between subgenomes, such as that in the middle regions of PseC-chr10 and PsoC-chr10, are inferred from inconsistencies between subgenome assignments calculated using chromosomes (ring a) and windows (rings b–d).DThe mapping depth of Illumina sequencing reads fromP. somniferumtoP. setigerumsubgenomes.EInsertion times of subgenome-specific LTR-RTs. The 95% confidence intervals (CI) of the insertion times are used to infer the time boundary of divergence to hybridization period. 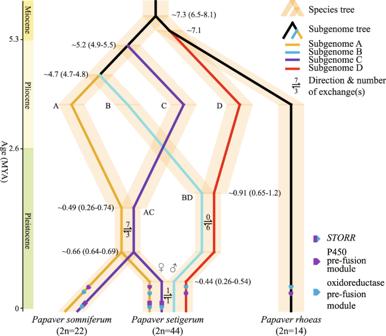Fig. 2: The reticulate allopolyploidization model in the threePapaverspecies and the subgenomic locations ofSTORRand its pre-fusion loci. The times of species/subgenomes divergence and hybridization shown on the topology were based on medianKs values and the subgenome-specific LTR-RT insertion times, respectively, see Supplementary Tables3,4for details. The currently retained copies ofSTORRand its pre-fusion modules are sorted to subgenomes (see more details in Supplementary Figs.13–15). Purple and blue denote the cytochrome P450 and oxidoreductase modules, respectively, to correspond with the scheme of Fig. 3a in Yang et al.3. Reconstruction of gene and macro-synteny trees for the three studied Papaver species Syntenic blocks within the three Papaver species were identified with OrthoFinder v2.3.1 [5] . Orthologous and paralogous relationships, as well as orthogroups, were inferred using the parameters “-M msa -T fasttree” based on proteome sequences from multiple species. The resulting gene pairs were used to call collinear/syntenic blocks using MCScanX (parameters: -a -b 0 -c 0) [6] . For syntenic homologous gene pairs, K s was calculated using the ParaAT pipeline [13] (Supplementary Figs. 2 – 3 ). Briefly, the protein sequences of each gene pair were first aligned in MUSCLE v3.8.425 [14] , and the alignment was then converted to a codon alignment using PAL2NAL v14 [15] . The K s was finally calculated using KaKs_Calculator v2.0 [16] with the YN model [17] . We then extracted 4,791 anchor genes from the inter-genomic syntenic blocks in P. rhoeas , P. somniferum and P. setigerum with a ratio of exactly 1:2:4. To reconstruct the gene trees, the homoeologous gene sequences were aligned with MAFFT v7.481 [18] and trimmed with trimAl v1.2 [19] using a heuristic selection optimized for maximum likelihood (ML) phylogenetic tree reconstruction. Then, the ML tree (Supplementary Fig. 4 ) was inferred using IQ-TREE v1.6.12 [7] with 1000 bootstraps [20] . The 1:2:4 genes located on the same chromosome set were considered as macro-synteny, and two methods were used to infer the macro-synteny trees (Supplementary Fig. 5 ): the ML and the coalescence-based method. For the ML method, the gene alignments generated earlier were concatenated, and a tree was reconstructed using IQ-TREE [7] with 1000 bootstraps [20] . For the coalescence-based method, the gene trees were input into ASTRAL (MP-5.14.5) [11] to infer the tree based on coalescence. Phasing the subgenomes of P. somniferum and P. setigerum , and inference of species/subgenome trees We used SubPhaser (parameters: -q 150 -exclude_exchanges) [4] to phase and partition the subgenomes of P. somniferum and P. setigerum (Supplementary Figs. 6 – 7 ). In brief, chromosomes of a neoallopolyploid were assigned to subgenomes based on differential repetitive k- mers that were assumed to have expanded during the period of independent evolution after divergence from the nearest common ancestor and before the hybridization of the parental progenitors (the so-called divergence–hybridization period). A subgenome is considered to be well-phased when it displays distinct patterns of both differential k -mers and homoeologous chromosomes, confirming the presence of subgenome-specific features, as expected. We considered each subgenome as an independent pseudo-species for the subsequent phylogenomic analyses. We additionally collected genomic data from 15 other taxa in the Ranunculales and other angiosperm lineages, as well as RNA-Seq data from P. bracteatum , from published papers and public databases (see Data Availability for details). The transcriptome of P. bracteatum was first de novo assembled using Trinity v2.6.6 [21] and the coding region of each transcript was annotated using TransDecoder v5.2.0 ( https://github.com/TransDecoder/TransDecoder/ ). Only transcripts with the longest coding region for each gene were retained, and only genes with complete coding regions were used for downstream analyses. We inferred orthogroups from these data using OrthoFinder v2.3.1 [5] as described above. Finally, we inferred the species/subgenome trees (Supplementary Fig. 8 ) using both ML and coalescence-based methods, as described earlier. Identification and validation of exchanges between subgenomes The identification of exchanges between subgenomes (Supplementary Figs. 6 – 7 , Fig. 1C ) was carried out using SubPhaser [4] in a semi-automated process. SubPhaser assigned each 1 Mb genomic window to subgenomes and flagged windows with enrichments that did not match the subgenome assignments of their chromosome as potential exchanges. These were further checked manually to determine whether they were bona fide exchanges or not. For example, in the middle of C-Pse-chr10 (Supplementary Fig. 6D ), subgenome A-specific k- mers showed continuous significant enrichments (2nd circle from outer to inner circles), and the abundance of subgenome A-specific k- mers was comparable to those on subgenome A chromosomes (4th circle) which contrasted with the other subgenomes (5–7th circles). Based on these observations, we confidently concluded that an exchange had occurred. After manually checking, we excluded short exchanges with lengths of less than 5 Mb (Supplementary Tables 1 – 2 ). As unbalanced exchanges were expected to have syntenic blocks within subgenomes, we validated them through syntenic analyses (Supplementary Figs. 2 – 3 ). For example, we observed an exchange where the segment at the 5ʹ end of PseC-15 had been exchanged to the 3ʹ end of PseB-17, resulting in a large syntenic block between PseB-17-3’ and naive PsoB-5-5’ (Supplementary Fig. 2 ). Due to this imbalance, subgenome PseB now has two copies of this homoeologous segment, leading to a large syntenic block between PseB-17-3’ and PseB-13-3’ where the PseB-naive homoeologous segment is located (Supplementary Fig. 3 ). Comparison of genomic composition of P. somniferum and P. setigerum We used the sppIDer [8] pipeline to confirm the genomic composition of P. somniferum and P. setigerum (Fig. 1D ). This involved mapping short-read sequencing data from P. somniferum to the genome of P. setigerum to assess the genomic contribution and relative ploidy of each of the subgenomes. Identification of potential progenitor species with other Papaver species To identify potential progenitor species, all available sequencing data (i.e. the genome skimming data) from Papaver species were downloaded from public databases (see Data Availability for details). The genome skimming data were assembled using the HybPiper pipeline [10] , where the short sequencing reads were mapped to each homologous gene group using BWA-MEM v0.7.17 [22] , and assembled with SPAdes v3.13.1 [23] . The coding regions were then annotated with exonerate v2.2.0 [24] . A total of 1474 single-copy genes were extracted, and a species tree (Supplementary Fig. 9 ) was inferred using methods described above. P. dubium has the potential to be the tetraploid progenitor (BD) of P. setigerum . To explore this possibility further, we downloaded the transcript sequences of P. dubium subsp. lecoqii from a recent study [12] and annotated the coding regions using TransDecoder v5.2.0. Next, we inferred orthogroups with OrthoFinder v2.3.1 [5] and calculated Ks for both orthologous and paralogous gene pairs using the ParaAT pipeline [13] . Using the K s-based method, we inferred potential recent WGD events in P. dubium subsp. lecoqii (Supplementary Fig. 10 ). Identification of potential maternal parent using the chloroplast tree To determine the potential maternal parent of P. somniferum and P. setigerum , we assembled chloroplast genomes from short-read sequencing data of Papaver species using GetOrganelle v1.6.2e (parameters: -w 115 -R 13) [25] . The assembled genomes were then annotated using the OGAP pipeline ( https://github.com/zhangrengang/ogap ). Based on whole plastome sequences of Papaver and related taxa, a phylogenomic tree (Supplementary Fig. 11 ) was inferred using IQ-TREE [7] with 1000 bootstraps [20] . Estimation of divergence and hybridization times The timing of species/subgenome divergence and hybridization (Supplementary Tables 3 – 4 , Supplementary Figs. 6 – 7 , Fig. 1E ) were estimated with two methods: the LTR-based method and the K s-based method. Subgenome-specific long terminal repeat retrotransposons (LTR-RTs) are expected to undergo a burst of activity during the divergence–hybridization period. We employed SubPhaser, which uses subgenome-specific LTR-RTs to estimate the upper and lower boundaries of the divergence–hybridization period by applying a symmetric 95% percentile-based confidence interval to the subgenome-specific LTR insertion ages. The analysis excluded any potential exchanged LTR-RTs. Due to the large uncertainty in time estimation using LTR-RTs (particularly for the divergence time) [4] , a traditional K s-based method [3] was also used to estimate the divergence time independently, based on a divergence time of P. somniferum–P. rhoeas (7.7 MYA [3] ). The estimated times were calculated using the formula 1 : 
    T=Ks/Ks(P.somniferum-P.rhoeas)*7.7 MYA
 (1) assuming an equal substitution rate per year. Assignment of subgenome and building gene phylogenies for STORR -related loci Subgenomes for STORR -related loci (Supplementary Figs. 13 – 15 , Fig. 2 ) were determined by their locations on subgenome segments (Supplementary Tables 1 – 2 ) using bedtools v2.27.1 [26] . Gene trees (Supplementary Figs. 13 – 14 ) were reconstructed using IQ-TREE [7] with 1000 bootstraps [20] . Reporting summary Further information on research design is available in the Nature Portfolio Reporting Summary linked to this article.